Connexin40 regulates platelet function The presence of multiple connexins was recently demonstrated in platelets, with notable expression of Cx37. Studies with Cx37-deficient mice and connexin inhibitors established roles for hemichannels and gap junctions in platelet function. It was uncertain, however, whether Cx37 functions alone or in collaboration with other family members through heteromeric interactions in regulation of platelet function. Here we report the presence and functions of an additional platelet connexin, Cx40. Inhibition of Cx40 in human platelets or its deletion in mice reduces platelet aggregation, fibrinogen binding, granule secretion and clot retraction. The effects of the Cx37 inhibitor 37,43 Gap27 on Cx40 −/− mouse platelets and of the Cx40 inhibitor 40 Gap27 on Cx37 −/− mouse platelets revealed that each connexin is able to function independently. Inhibition or deletion of Cx40 reduces haemostatic responses in mice, indicating the physiological importance of this protein in platelets. We conclude that multiple connexins are involved in regulating platelet function, thereby contributing to haemostasis and thrombosis. Connexins are a family of membrane proteins that assemble into connexons or hemichannels on the plasma membrane by oligomerization of six connexin monomers [1] . Hemichannels facilitate the transport of small molecules (up to ~1,000 Da) between the interior and exterior of isolated cells [2] , [3] and form gap junctions on docking of connexons between adjacent cells, allowing direct intercellular communication [1] . Over 20 connexins have been identified in various mammalian cell types, which are capable of forming homomeric (that is comprising a single connexin type) or heteromeric (that is comprising more than one connexin type) hemichannels and gap junctions with varying conductance properties [4] , [5] , [6] , [7] , [8] . Gap junction-mediated intercellular communication has vital roles in several cell types and tissues such as nerve cells [9] , bone marrow stromal cells [10] , oocytes [11] and cardiac muscle [12] , and recent studies have identified roles for connexins in circulating cells such as monocytes [13] , T-cells [14] , [15] and platelets [16] , [17] . Platelets aggregate on vessel wall damage to prevent bleeding at the site of injury [18] . We recently reported [17] the presence of multiple connexins in platelets with notable expression of Cx37. The study demonstrated gap junction-dependent intercellular communication between platelets and a role for connexin hemichannels and gap junctions in platelet function [17] . Gap junction blockers such as carbenoxolone, 18β-glycyrrhetinic acid and 37,43 Gap27 (refs 19 , 20 ), with varying selectivity, reduced a range of platelet functions including aggregation and clot retraction [17] . It is uncertain, however, whether other connexin family members are involved, and a recent study suggested Cx37 alone to be present and functional in platelets [16] . Given the possibility of heteromeric hemichannel formation, these connexins may depend on each other to elicit their functions. In this report we demonstrate the presence of another vascular connexin, Cx40, in platelets. We show that Cx40 and Cx37 are able to function independently of each other in platelets, and establish that multiple connexin family members contribute to the promotion of haemostasis. Inhibition of Cx40 reduces platelet activation Transcriptomic analysis revealed Cx40 to be expressed in megakaryocytes [17] . In the present study we confirmed the presence of Cx40 protein in human platelets ( Fig. 1a and Supplementary Fig. S1 ), the levels of which were unaltered following stimulation of platelets with a glycoprotein (GP) VI-selective (collagen receptor) ligand, cross-linked collagen-related peptide (CRP-XL). The effect of 40 Gap27 (ref. 19 ), a selective Cx40 mimetic peptide inhibitor (this peptide comprises an 11-amino-acid residue sequence mimicking a region of extracellular loop and that can competitively prevent gap-junction formation or interfere with hemichannel function) on human platelet aggregation was explored. Washed human platelets were stimulated with CRP-XL in the presence of increasing concentrations of 40 Gap27. Aggregation induced by CRP-XL (0.5 μg ml −1 ) was reduced by ~50%, 35% and 15% at 100, 50 and 10 μg ml −1 of 40 Gap27, respectively ( Fig. 1b,c ). The reduction in aggregation was less pronounced (20% inhibition with 100 μg ml −1 of 40 Gap27) when a higher CRP-XL concentration (1 μg ml −1 ) was used ( Fig. 1d,e ). A scrambled peptide control for 40 Gap27 showed no effect ( Fig. 1f,g ). Cx40 involvement in the regulation of platelet function was not restricted to GPVI-mediated activation, as thrombin- (0.1 U ml −1 ; Fig. 1h,i ) and ADP- (10 μM; Fig. 1j,k ) induced aggregation was also inhibited by 40 Gap27. This is consistent with the inability of connexins to modulate GPVI-proximal signalling events [17] . 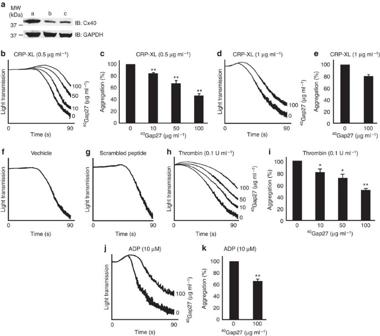Figure 1: Presence of Cx40 and effects of its inhibition on platelet function. (a) Presence of Cx40 in human platelets was confirmed by immunoblot analysis (human umbilical vascular endothelial cells (a), and resting (b) or CRP-XL- (1 μg ml−1) stimulated human platelets (c)). Glyceraldehyde 3-phosphate dehydrogenase (GAPDH) was detected as a loading control. Human platelet aggregation performed in the presence or absence of40Gap27 was recorded for 90 s following stimulation with 0.5 (b,c) or 1 μg ml−1(d,e) CRP-XL (a scrambled peptide control showed no effect on aggregation compared with the vehicle (f,g)), 0.1 U ml−1thrombin (h,i) and 10 μM ADP (j,k). Cumulative data represent mean±s.d. (n=4). The level of aggregation obtained with vehicle was taken as 100% (Student’st-test, *P<0.05 and **P<0.01). Figure 1: Presence of Cx40 and effects of its inhibition on platelet function. ( a ) Presence of Cx40 in human platelets was confirmed by immunoblot analysis (human umbilical vascular endothelial cells ( a ), and resting ( b ) or CRP-XL- (1 μg ml −1 ) stimulated human platelets ( c )). Glyceraldehyde 3-phosphate dehydrogenase (GAPDH) was detected as a loading control. Human platelet aggregation performed in the presence or absence of 40 Gap27 was recorded for 90 s following stimulation with 0.5 ( b , c ) or 1 μg ml −1 ( d , e ) CRP-XL (a scrambled peptide control showed no effect on aggregation compared with the vehicle ( f , g )), 0.1 U ml −1 thrombin ( h , i ) and 10 μM ADP ( j , k ). Cumulative data represent mean±s.d. ( n =4). The level of aggregation obtained with vehicle was taken as 100% (Student’s t -test, * P <0.05 and ** P <0.01). Full size image Deletion of Cx40 reduces platelet activation To further assess the importance of Cx40 in platelet function, Cx40 −/− mouse platelets were examined. Immunoblot analysis confirmed the absence of Cx40 in platelets ( Fig. 2a ). To exclude compensatory effects of Cx40 deletion on expression of other family members, the levels of other platelet connexins, such as Cx32 ( Fig. 2b ), Cx37 ( Fig. 2c ) and Cx43 ( Fig. 2d ), were analysed in Cx40 −/− platelets by immunoblot analysis and were indistinguishable from those in Cx40 +/+ platelets. Expression levels of platelet receptors: integrins αIIbβ3 ( Fig. 2e ), α 2 β 1 ( Fig. 2f ), GPVI ( Fig. 2g ) and GPIb ( Fig. 2h ) on Cx40 −/− and Cx40 +/+ platelets were found to be similar. 40 Gap27 (100 μg ml −1 ) inhibited CRP-XL- (0.5 μg ml −1 ) stimulated mouse ( Cx40 +/+ ) platelet aggregation by ~30% ( Fig. 2i ) but exhibited no inhibitory effects on Cx40 −/− platelets ( Fig. 2j ), confirming inhibitor selectivity. CRP-XL- (0.5 μg ml −1 ) induced aggregation was reduced by around 50% in Cx40 −/− platelets compared with Cx40 +/+ platelets ( Fig. 2k,l ), with slightly less-pronounced inhibition (30% inhibition) at higher agonist concentrations (for example, 1 μg ml −1 CRP-XL; Fig. 2m,n ). 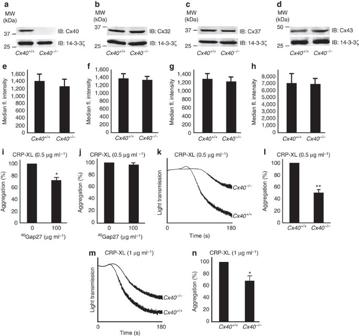Figure 2: Deletion ofCx40affects platelet activation. Deletion ofCx40was confirmed inCx40−/−mouse platelets by immunoblotting (a). The expression ofCx32(b),Cx37(c) andCx43(d) were analysed by immunoblot analysis usingCx40+/+andCx40−/−mouse platelets. 14-3-3ζ was detected as a loading control. Blots are representative of four separate experiments. The expression levels of αIIbβ3 (e), α2β1(f), GPVI (g) and GPIbα (h) were analysed onCx40+/+andCx40−/−mouse platelets by flow cytometry. Platelet aggregation performed in the presence or absence of40Gap27 using washed platelets obtained fromCx40+/+(i) andCx40−/−(j) mice was recorded for 180 s following stimulation with CRP-XL (0.5 μg ml−1). The level of aggregation obtained in the absence of40Gap27 was taken as 100%. Similar aggregations were performed using washed platelets obtained fromCx40+/+andCx40−/−mice following stimulation with 0.5 (k,l) or 1 μg ml−1CRP-XL (m,n). Data represent mean±s.d. (n=4). The level of aggregation obtained withCx40+/+was taken as 100% (Student’st-test, *P<0.05 and **P<0.01). Figure 2: Deletion of Cx40 affects platelet activation. Deletion of Cx40 was confirmed in Cx40 −/− mouse platelets by immunoblotting ( a ). The expression of Cx32 ( b ), Cx37 ( c ) and Cx43 ( d ) were analysed by immunoblot analysis using Cx40 +/+ and Cx40 −/− mouse platelets. 14-3-3ζ was detected as a loading control. Blots are representative of four separate experiments. The expression levels of αIIbβ3 ( e ), α 2 β 1 ( f ), GPVI ( g ) and GPIbα ( h ) were analysed on Cx40 +/+ and Cx40 −/− mouse platelets by flow cytometry. Platelet aggregation performed in the presence or absence of 40 Gap27 using washed platelets obtained from Cx40 +/+ ( i ) and Cx40 −/− ( j ) mice was recorded for 180 s following stimulation with CRP-XL (0.5 μg ml −1 ). The level of aggregation obtained in the absence of 40 Gap27 was taken as 100%. Similar aggregations were performed using washed platelets obtained from Cx40 +/+ and Cx40 −/− mice following stimulation with 0.5 ( k , l ) or 1 μg ml −1 CRP-XL ( m , n ). Data represent mean±s.d. ( n =4). The level of aggregation obtained with Cx40 +/+ was taken as 100% (Student’s t -test, * P <0.05 and ** P <0.01). Full size image Cx40 modulates inside-out signalling to integrin αIIbβ3 The inhibition of platelet aggregation in response to 1 μg ml −1 CRP-XL following Cx40 blockade was accompanied by reduced fibrinogen binding (60% decrease with 100 μg ml −1 of 40 Gap27), indicating the involvement of this connexin in platelet inside-out signalling to integrin αIIbβ3 ( Fig. 3a ). The inhibitory effects of 40 Gap27 were also observed when human platelets were stimulated with ADP (10 μM; Fig. 3b ) or thrombin (0.1 U ml −1 ; Fig. 3c ). Similarly, fibrinogen binding to CRP-XL- (1 μg ml −1 ) stimulated mouse platelets in whole blood was reduced by ~50% in Cx40 −/− platelets compared with Cx40 +/+ platelets ( Fig. 3d ). 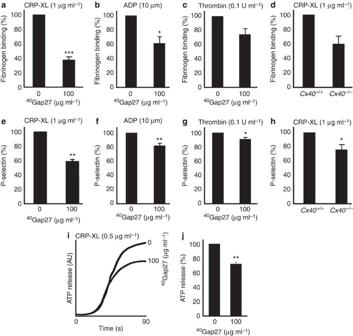Figure 3: Inhibition or deletion of Cx40 reduces platelet inside-out signalling and granule secretion. The effect of40Gap27 on 1 μg ml−1CRP-XL- (a), 10 μM ADP- (b) and 0.1 U ml−1thrombin- (c) induced fibrinogen binding was measured by flow cytometry using human PRP. Similarly, fibrinogen binding toCx40+/+andCx40−/−mouse platelets was measured using whole blood following stimulation with 1 μg ml−1CRP-XL (d). Fibrinogen binding obtained with vehicle orCx40+/+was taken as 100%. Human PRP was stimulated with 1 μg ml−1CRP-XL (e), 10 μM ADP (f) and 0.1 U ml−1thrombin (g) in the presence and absence of40Gap27 (100 μg ml−1) and the level of P-selectin exposed on surface measured by flow cytometry. Similarly, P-Selectin exposure upon stimulation with 1 μg ml−1CRP-XL using whole blood obtained fromCx40+/+andCx40−/−was measured (h). P-selectin exposure with vehicle orCx40+/+was taken as 100%. Human washed platelets were stimulated with 0.5 μg ml−1CRP-XL in the presence and absence of40Gap27 (100 μg ml−1), and the level of ATP secretion was measured using lumino-aggregometry (i,j). Data represent mean±s.d. (n=4; Student’st-test, *P<0.05, **P<0.01 and ***P<0.001). Figure 3: Inhibition or deletion of Cx40 reduces platelet inside-out signalling and granule secretion. The effect of 40 Gap27 on 1 μg ml −1 CRP-XL- ( a ), 10 μM ADP- ( b ) and 0.1 U ml −1 thrombin- ( c ) induced fibrinogen binding was measured by flow cytometry using human PRP. Similarly, fibrinogen binding to Cx40 +/+ and Cx40 −/− mouse platelets was measured using whole blood following stimulation with 1 μg ml −1 CRP-XL ( d ). Fibrinogen binding obtained with vehicle or Cx40 +/+ was taken as 100%. Human PRP was stimulated with 1 μg ml −1 CRP-XL ( e ), 10 μM ADP ( f ) and 0.1 U ml −1 thrombin ( g ) in the presence and absence of 40 Gap27 (100 μg ml −1 ) and the level of P-selectin exposed on surface measured by flow cytometry. Similarly, P-Selectin exposure upon stimulation with 1 μg ml −1 CRP-XL using whole blood obtained from Cx40 +/+ and Cx40 −/− was measured ( h ). P-selectin exposure with vehicle or Cx40 +/+ was taken as 100%. Human washed platelets were stimulated with 0.5 μg ml −1 CRP-XL in the presence and absence of 40 Gap27 (100 μg ml −1 ), and the level of ATP secretion was measured using lumino-aggregometry ( i , j ). Data represent mean±s.d. ( n =4; Student’s t -test, * P <0.05, ** P <0.01 and *** P <0.001). Full size image Inhibition or deletion of Cx40 affects platelet secretion The level of P-selectin exposed on the surface of platelets (a marker for α-granule secretion) following stimulation with CRP-XL (1 μg ml −1 ) was measured in the presence or absence of 40 Gap27 (100 μg ml −1 ) using human platelet-rich plasma (PRP). This was reduced by ~40% in the presence of 40 Gap27 (100 μg ml −1 ; Fig. 3e ). Reduced platelet granule secretion was also observed upon stimulation of human platelets with ADP (10 μM; Fig. 3f ) or thrombin (0.1 U ml −1 ; Fig. 3g ). Similarly, P-selectin exposure on Cx40 −/− mouse platelets was reduced upon stimulation with 1 μg ml −1 CRP-XL in comparison with Cx40 +/+ mouse platelets ( Fig. 3h ). The observed effects of Cx40 inhibition or deletion on individual platelets analysed by flow cytometry (fibrinogen binding and P-selectin exposure; Fig. 3a–h ) point towards the importance of Cx40 hemichannels in platelet activation. To assess the effects of Cx40 inhibition on dense granule secretion, the consequences of 40 Gap27 treatment of human washed platelets on ATP secretion was assessed. CRP-XL (0.5 μg ml −1 ) induced ATP release was inhibited by ~40% with 40 Gap27 (100 μg ml −1 ; Fig. 3i,j ). Together, these data suggest that Cx40 has an important role in granule secretion. The effects of Cx40 are not solely secretion dependent To assess whether diminished platelet activation during Cx40 blockade is due solely to the reduced levels of granule secretion and secondary activators of platelet function, CRP-XL-induced fibrinogen binding was measured in the presence of apyrase, an enzyme that hydrolyses the ADP and the TXA 2 synthesis blocker indomethacin (through inhibition of cyclooxygenase). Addition of a saturating concentration of apyrase (4 U ml −1 ) in PRP reduced the fibrinogen binding to 70% when stimulated with CRP-XL (0.5 μg ml −1 ; Fig. 4a ). Similarly, addition of indomethacin at a saturating concentration of 20 μM reduced the fibrinogen binding by ~80% upon CRP-XL (0.5 μg ml −1 ) stimulation ( Fig. 4a ). The addition of both apyrase (4 U ml −1 ) and indomethacin (20 μM) reduced the fibrinogen binding level by ~85% with CRP-XL (0.5 μg ml −1 ; Fig. 4a ). An increased concentration of CRP-XL (1 μg ml −1 ) resulted in a similar level of inhibition at the same concentration of apyrase and indomethacin ( Fig. 4b ). Addition of 40 Gap27 (100 μg ml −1 ) along with 4 U ml −1 apyrase or 20 μM indomethacin or both, resulted in a further reduction in fibrinogen-binding levels ( Fig. 4c,d ) at lower and higher concentration of CRP-XL, indicating that the inhibitory effects of 40 Gap27 on platelet functions are not solely due to defects in secreted ADP or the synthesis of TXA 2 . Consistent with these data, the inhibition of Cx40 or Cx37 with 40 Gap27 or 37,43 Gap27 (100 μg ml −1 ), respectively, or the deletion of either connexin in mouse platelets did not affect the level of TXB 2 (a stable TXA 2 metabolite) synthesized in platelets after platelet activation by CRP-XL ( Fig. 5 ). 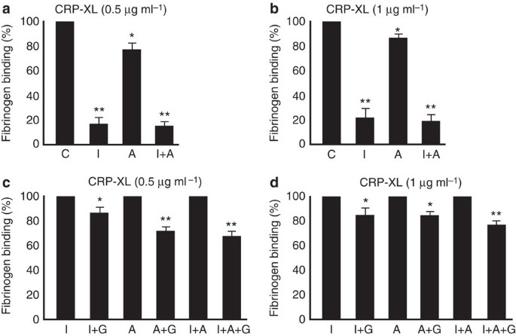Figure 4: Inhibitory effects of40Gap27 on platelet function are not solely due to defects in granule secretion or TXA2synthesis. The level of fibrinogen binding was measured in the presence and absence of apyrase (4 U ml−1) or indomethacin (20 μM), or both (at the same concentration) on 0.5 (a) and 1 μg ml−1(b) CRP-XL activation in human PRP. The level of fibrinogen binding obtained in the absence of apyrase or indomethacin was taken as 100%. Similarly, 0.5 (c) and 1 μg ml−1(d) CRP-XL-induced fibrinogen binding was measured in the presence or absence of40Gap27 (100 μg ml−1) in addition to apyrase (4 U ml−1) and/or indomethacin (20 μM). The level of fibrinogen binding obtained in the absence of40Gap27 (but in the presence of apyrase and/or indomethacin) was taken as 100% to compare the inhibitory levels obtained with40Gap27. Data represent mean±s.d. (n=3; Student’st-test, *P<0.05 and **P<0.01). A, apyrase; C, control; G,40Gap27; I, indomethacin. Figure 4: Inhibitory effects of 40 Gap27 on platelet function are not solely due to defects in granule secretion or TXA 2 synthesis. The level of fibrinogen binding was measured in the presence and absence of apyrase (4 U ml −1 ) or indomethacin (20 μM), or both (at the same concentration) on 0.5 ( a ) and 1 μg ml −1 ( b ) CRP-XL activation in human PRP. The level of fibrinogen binding obtained in the absence of apyrase or indomethacin was taken as 100%. Similarly, 0.5 ( c ) and 1 μg ml −1 ( d ) CRP-XL-induced fibrinogen binding was measured in the presence or absence of 40 Gap27 (100 μg ml −1 ) in addition to apyrase (4 U ml −1 ) and/or indomethacin (20 μM). The level of fibrinogen binding obtained in the absence of 40 Gap27 (but in the presence of apyrase and/or indomethacin) was taken as 100% to compare the inhibitory levels obtained with 40 Gap27. Data represent mean±s.d. ( n=3 ; Student’s t -test, * P <0.05 and ** P <0.01). A, apyrase; C, control; G, 40 Gap27; I, indomethacin. 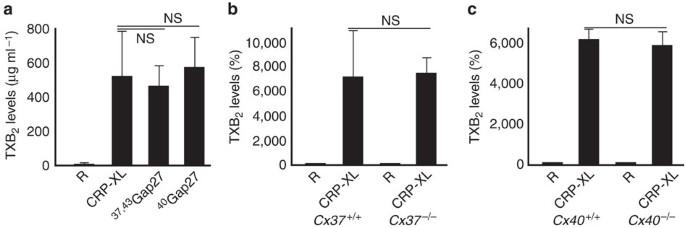Figure 5: Inhibition or deletion of Cx40 or Cx37 does not affect TXB2synthesis in platelets. The levels of TXB2were measured by immunoassay in human PRP following stimulation with 1 μg ml−1CRP-XL in the presence or absence of 100 μg ml−1of40Gap27 or37,43Gap27 (a). Similarly, TXB2levels were measured inCx37−/−(b) andCx40−/−(c) mouse platelets upon stimulation with 1 μg ml−1CRP-XL. The levels of TXB2obtained in human platelets were shown as concentrations. The levels of TXB2obtained with resting platelets inCx37+/+orCx40+/+mouse platelets were taken as 100% for comparison withCx37-orCx40-deficient mouse platelets. R, resting platelets. Data represent mean±s.d. (n=3; Student’st-test was used for statistical analysis). Full size image Figure 5: Inhibition or deletion of Cx40 or Cx37 does not affect TXB 2 synthesis in platelets. The levels of TXB 2 were measured by immunoassay in human PRP following stimulation with 1 μg ml −1 CRP-XL in the presence or absence of 100 μg ml −1 of 40 Gap27 or 37,43 Gap27 ( a ). Similarly, TXB 2 levels were measured in Cx37 −/− ( b ) and Cx40 −/− ( c ) mouse platelets upon stimulation with 1 μg ml −1 CRP-XL. The levels of TXB 2 obtained in human platelets were shown as concentrations. The levels of TXB 2 obtained with resting platelets in Cx37 +/+ or Cx40 +/+ mouse platelets were taken as 100% for comparison with Cx37- or Cx40 -deficient mouse platelets. R, resting platelets. Data represent mean±s.d. ( n=3 ; Student’s t -test was used for statistical analysis). Full size image Cx40 functions independently from Cx37 As connexins may form homomeric or heteromeric hemichannels, we sought to determine whether Cx40 and Cx37 function independently on platelets. The specificity of action of 40 Gap27 or 37,43 Gap27 was first confirmed to establish a lack of inhibitory effect on Cx40- and Cx37-deficient mouse platelets, respectively ( Fig. 2j and Fig. 6a,b ,). 40 Gap27 (100 μg ml −1 ) inhibited CRP-XL-stimulated (1 μg ml −1 ) fibrinogen binding ( Fig. 7a ) and P-selectin exposure ( Fig. 7b ) in Cx37 −/− mouse platelets to a similar extent to that observed in Cx37 +/+ platelets. Similarly, 37,43 Gap27 (100 μg ml −1 ) inhibited fibrinogen binding ( Fig. 7c ) and P-selectin exposure ( Fig. 7d ) in Cx40 −/− mouse platelets to a similar level as that observed on Cx40 +/+ platelets. Together, these data demonstrate that both Cx37 and Cx40 are able to contribute to platelet regulation independently. 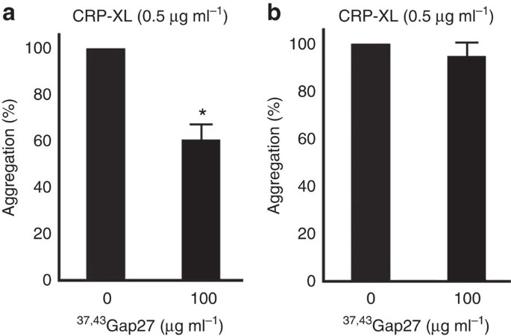Figure 6:37,43Gap27 does not affectCx37>−/−platelets confirming its selectivity. Platelet aggregation performed in the presence or absence of37,43Gap27 (100 μg ml−1) using washed platelets obtained fromCx37+/+(a) andCx37−/−(b) mice was recorded for 180 s following stimulation with CRP-XL (0.5 μg ml−1). The level of aggregation obtained in the absence of37,43Gap27 was taken as 100%. Data represent mean±s.d. (n=3; Student’st-test, *P<0.05). Figure 6: 37,43 Gap27 does not affect Cx37> −/− platelets confirming its selectivity. Platelet aggregation performed in the presence or absence of 37,43 Gap27 (100 μg ml −1 ) using washed platelets obtained from Cx37 +/+ ( a ) and Cx37 −/− ( b ) mice was recorded for 180 s following stimulation with CRP-XL (0.5 μg ml −1 ). The level of aggregation obtained in the absence of 37,43 Gap27 was taken as 100%. Data represent mean±s.d. ( n =3; Student’s t -test, * P <0.05). 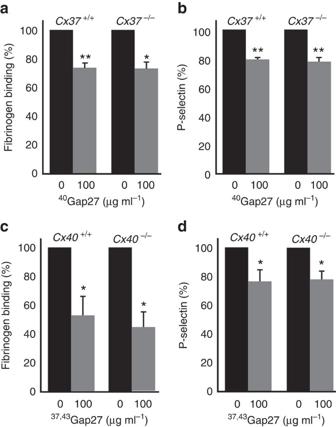Figure 7: Cx40 regulates platelet function independently from Cx37. The levels of fibrinogen binding (a) and P-selectin exposure (b) inCx37+/+andCx37−/−mouse platelets in the presence or absence of40Gap27 (100 μg ml−1) were measured by flow cytometry using whole blood following stimulation with 1 μg ml−1CRP-XL. Similarly, the levels of fibrinogen binding (c) and P-selectin exposure (d) inCx40+/+andCx40−/−mouse platelets in the presence or absence of37,43Gap27 (100 μg ml−1) were measured following stimulation with 1 μg ml−1CRP-XL. The level of fibrinogen binding obtained in the absence of inhibitor was taken 100%. Data represent mean±s.d. (n=4; Student’st-test, *P<0.05 and **P<0.01). Full size image Figure 7: Cx40 regulates platelet function independently from Cx37. The levels of fibrinogen binding ( a ) and P-selectin exposure ( b ) in Cx37 +/+ and Cx37 −/− mouse platelets in the presence or absence of 40 Gap27 (100 μg ml −1 ) were measured by flow cytometry using whole blood following stimulation with 1 μg ml −1 CRP-XL. Similarly, the levels of fibrinogen binding ( c ) and P-selectin exposure ( d ) in Cx40 +/+ and Cx40 −/− mouse platelets in the presence or absence of 37,43 Gap27 (100 μg ml −1 ) were measured following stimulation with 1 μg ml −1 CRP-XL. The level of fibrinogen binding obtained in the absence of inhibitor was taken 100%. Data represent mean±s.d. ( n=4 ; Student’s t -test, * P <0.05 and ** P <0.01). Full size image Cx40 is important for clot retraction We have shown previously that gap junctions contribute to intercellular communication and the coordination of clot retraction [17] . As observed for general gap-junction blockers and 37,43 Gap27 (ref. 17 ), 40 Gap27 did not alter the initial clot formation but reduced clot retraction threefold at 90 min ( Fig. 8a,b ). Clot retraction was reduced to a similar extent in Cx40 −/− compared with Cx40 +/+ mouse platelets ( Fig. 8c,d ). These data suggest that inhibition of Cx40-mediated intercellular signalling reduces outside-in signalling through integrin αIIbβ3, which drives clot retraction. 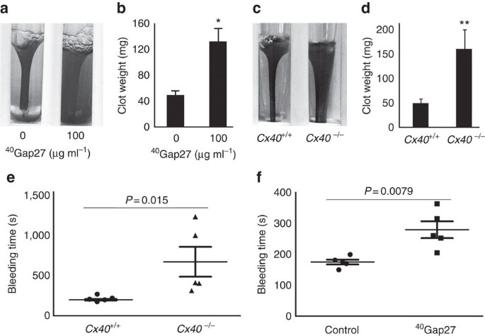Figure 8: Cx40 regulates clot retraction and haemostasis. The effect of40Gap27 on clot retraction using human PRP was analysedin vitrofor 90 min (a,b). The effect of Cx40 deficiency on clot retraction was analysed (c,d). Data represent mean±s.d. (n=4; Student’st-test, *P<0.05 and **P<0.01). Deletion of Cx40 or the effect of40Gap27 (estimated plasma concentration: 100 μg ml−1) on haemostasis in mice was analysed by measuring the bleeding time after tail tip excision. The bleeding time obtained withCx40−/−mice were compared withCx40+/+mice (e). Similarly, the bleeding time obtained with scrambled peptide- (estimated 100 μg ml-1) treated group was compared with40Gap27-treated mice (f). Data represent mean±s.d. (n=5 forCx40+/+orCx40−/−mice andn=5 mice for scrambled peptide control or40Gap27 treated). The significance between control and treated groups, andP-values (as shown) were calculated by non-parametric Mann–Whitney test using GraphPad Prism. Figure 8: Cx40 regulates clot retraction and haemostasis. The effect of 40 Gap27 on clot retraction using human PRP was analysed in vitro for 90 min ( a , b ). The effect of Cx40 deficiency on clot retraction was analysed ( c , d ). Data represent mean±s.d. ( n =4; Student’s t -test, * P <0.05 and ** P <0.01). Deletion of Cx40 or the effect of 40 Gap27 (estimated plasma concentration: 100 μg ml −1 ) on haemostasis in mice was analysed by measuring the bleeding time after tail tip excision. The bleeding time obtained with Cx40 −/− mice were compared with Cx40 +/+ mice ( e ). Similarly, the bleeding time obtained with scrambled peptide- (estimated 100 μg ml -1 ) treated group was compared with 40 Gap27-treated mice ( f ). Data represent mean±s.d. ( n =5 for Cx40 +/+ or Cx40 −/− mice and n =5 mice for scrambled peptide control or 40 Gap27 treated). The significance between control and treated groups, and P -values (as shown) were calculated by non-parametric Mann–Whitney test using GraphPad Prism. Full size image Cx40 regulates haemostasis in mice To analyse the physiological importance of Cx40 for haemostasis, tail-bleeding assays were performed on mice. Mice were anaesthetized intraperitoneally and tail tips were transected to observe the bleeding time. Cx40 +/+ mice bled for 199 s (between 175 and 219 s) compared with the Cx40 −/− mice that bled for 657 s (between 309 and 1,200 s; Fig. 8e ). Similarly, wild-type mice were treated either with scrambled control peptide or 40 Gap27 (at an estimated circulating concentration of 100 μg ml −1 ) for 3 min before transection of the tail tip. Control peptide-treated mice bled for 175 s (between 150 and 199 s), whereas 40 Gap27-treated mice bled for 279 s (between 205 and 363 s; Fig. 8f ). These data together suggest that Cx40 has a significant role in the maintenance of haemostasis. A previous study [16] described the presence of Cx37 as the only connexin expressed in platelets, where the effects of general inhibitors were attributed to the function of this connexin alone. We have, however, reported the presence of multiple connexins and the effects of non-selective connexin inhibitors and Cx37 deficiency on platelet function [17] . The present findings broaden the repertoire of platelet connexins that participate in platelet function to Cx40. Inhibition of Cx40 with a selective peptide inhibitor resulted in reduction in platelet functions such as fibrinogen binding, aggregation and granule secretion, similar to the effects observed with the inhibition of Cx37, indicating activatory roles for both Cx40 and Cx37 in platelet function. These conclusions are supported by similar observations using mouse platelets that lack either connexin. The inhibitory effects observed with 40 Gap27 in the presence of apyrase and indomethacin suggest that the effects of Cx40 blockade on platelet aggregation are not solely due to reduced granule secretion or TXA 2 synthesis. Further experiments using a Cx40 inhibitor on Cx37 −/− platelets and Cx37 inhibitor on Cx40 −/− platelets suggest that these connexins are able to function independently from each other. Consistent with this observation, we have failed to demonstrate heterotypic interactions between Cx40 and Cx37 through co-immunoprecipitation experiments. The inhibitory effects of 40 Gap27 on haemostasis, mirrored in the phenotype of Cx40 −/− mice, indicate the physiological importance of Cx40 in the maintenance of haemostasis. These data together with our previous study suggest that the hemichannels may have key roles in the initial activation of platelets when they are in isolation, although the nature of the signals conveyed by the hemichannels are yet to be established. We have previously demonstrated that within a platelet thrombus, gap junctions form between the cells, to enable sustained contact-dependent signalling to control thrombus stability and clot retraction [17] . It is possible, therefore, that following platelet stimulation, as aggregates begin to form, both hemichannel and gap junctions between platelets may be important, with the latter representing a new communication paradigm for the propagation of initial activatory signals between platelets. The roles of other platelet connexins such as Cx32 and Cx43 in platelet function remain to be explored. It is possible that these connexins may also control activatory mechanisms in platelet function working independently from each other, or in combination with other family members. Further work is required to determine the nature of hemichannel- and gap-junction-dependent signalling events that regulate platelet activation and clot retraction, and to determine whether connexins on platelets mediate functional interactions with other cells in the vasculature in health and disease. A priority will be to identify the nature of the signalling molecules that are conveyed by platelet hemichannels or gap junctions. Understanding of the molecular mechanisms that regulate their conductance will be crucial to explore therapeutic (anti-thrombotic) potential. Platelet preparation and aggregation Human platelet preparation and aggregation assays were performed using standard methods [17] , [21] , [22] . Briefly, blood was obtained from aspirin-free, healthy human volunteers with written informed consent as approved by the University of Reading Research Ethics Committee. PRP was prepared by centrifuging the blood for 20 min at 102 g at room temperature for flow cytometry assays. Washed platelets were prepared by further centrifuging the PRP with PGI 2 (125 ng ml −1 ) at 1,413 g for 10 min at room temperature and resuspended in modified Tyrodes-HEPES buffer (134 mM NaCl, 2.9 mM KCl, 0.34 mM Na 2 HPO 4 .12H 2 O, 12 mM NaHCO 3 , 20 mM HEPES and 1 mM MgCl 2 , pH 7.3) to the final density of 4 × 10 8 cells per ml for aggregation assays. Contaminating blood cells were counted by light microscopy and were mainly erythrocytes; leukocytes were rarely encountered with total cell contaminant level of <1 per 13,000 platelets. Aggregation assays were performed by light transmission aggregometry using CRP-XL (a selective agonist for platelet collagen receptor GPVI, from Professor R Farndale (University of Cambridge, UK)), thrombin or ADP (Sigma Aldrich, UK) in the presence or absence of various concentrations of gap-junction inhibitors. 37,43 Gap27 (SRPTEKTIFII; Sigma Aldrich) and 40 Gap27 (SRPTEKNVFIV; Anaspec, USA) were used as selective inhibitors for Cx37 and Cx40, respectively. Scrambled peptides IPFVESKRTVN and REKIITSFIPT were used as negative controls for 40 Gap27 and 37,43 Gap27, respectively. Dense granule secretion and immunoblotting ATP secretion assays were performed using luciferin–luciferase luminescence substrate (Chrono-log, USA) by luminescence aggregometry [17] . The level of ATP secreted from washed platelets on stimulation with agonists such as CRP-XL in the presence and absence of 40 Gap27 was measured by observing the level of luminescence liberated. SDS–PAGE and immunoblotting were performed using standard protocols [17] , [23] , [24] . Cx40 antibodies (used at a dilution of 1:1,000) were obtained from Chemicon, USA. Rabbit anti-human 14-3-3ζ (1:2,000) or GAPDH (glyceraldehyde 3-phosphate dehydrogenase; 1:1,000; Santa Cruz Biotechnology, USA) were used to detect 14-3-3ζ or GAPDH to ensure equivalent levels of protein loading in immunoblots. The secondary antibodies for immunoblotting: Cy5 goat anti-rabbit IgG (1:1,000) and Cy3 goat anti-mouse IgG (1:1,000) antibodies were obtained from Invitrogen, UK. Mouse blood collection and platelet preparation Colonies of Cx40 −/− (refs 25 , 26 ) and Cx37 −/− (refs 27 , 28 ) mice were maintained on a C57BL6 genetic background, and littermate controls were used in all experiments. All animals were used following approval from the University of Reading Local Ethics Review Panel and license from the British Home Office. Mice were killed and the blood was collected immediately by cardiac puncture into a syringe containing ACD (2.5% sodium citrate, 2% D -glucose and 1.5% citric acid; at 1 (ACD):9 (blood) ratio) for aggregation assays. Similarly, the blood was collected into syringe containing 4% citrate (at 1 (citrate):9 (blood) ratio) for flow cytometry and clot retraction assays. The blood was centrifuged at 203 g for 8 min and PRP collected into fresh tubes. After addition of PGI 2 (12.5 ng ml −1 ), the PRP was further centrifuged at 1,028 g for 5 min. The resultant platelet pellet was resuspended in modified Tyrodes-HEPES buffer. The platelets were rested for 30 min before aggregation assays were performed. Flow cytometry CRP-XL-stimulated fibrinogen binding and P-selectin exposure were measured in human PRP using fluorescein isothiocyanate (FITC)-labelled rabbit anti-human fibrinogen antibodies (Dako UK Ltd) and mouse anti-human CD62P antibody (BD Biosciences, UK), respectively, in the presence or absence of different concentrations of respective inhibitors. Platelets were incubated with inhibitor or control for 3 min before activation with CRP-XL for 20 min at room temperature. The cells were then fixed in 0.2% (v/v) formyl saline before analysis by flow cytometry. Similarly, various receptor expression levels were measured on mouse platelets using FITC-conjugated antibodies for GPVI, integrin αIIbβ3, integrin α 2 β 1 and GPIbα obtained from Emfret Analytics (Germany). To measure the level of P-selectin exposure on mouse platelets, FITC-conjugated P-selectin antibody (Emfret Analytics) was used. Data were analysed by calculating the median fluorescence intensity. Clot retraction Human or mouse PRP (200 μl) was mixed with 5 μl of red blood cells, and vehicle or gap-junction inhibitor (as needed), and the final volume raised to 1 ml with modified Tyrodes-HEPES buffer. Fibrin clot formation was initiated by adding thrombin (1 U ml −1 ). Clot retraction around a glass capillary added before clot formation was observed over a period of 90 min at room temperature. Clot weight was measured as a marker for clot retraction at different time points. Assessment of haemostasis Experiments were performed in live mice with approval from the University of Reading Local Ethical Review Panel and British Home Office. C57BL/6 mice (7–8 weeks old; The Jackson Laboratory, UK) were anaesthetized using ketamine (80 mg kg −1 ) and xylazine (5 mg kg −1 ) administered via the intraperitoneal route 20 min before the experiment and placed on a heated mat. 40 Gap27 (estimated 100 μg ml −1 of blood based on the weight of mouse) or scrambled peptide control was injected via femoral vein 5 min before 1 mm of tail tip was removed using a scalpel blade, and the tail tip was placed in sterile saline at 37 °C. The time to cessation of bleeding was measured up to 10 min. Similarly, Cx40 +/+ and Cx40 −/− mice were anaesthetized and tail tip was removed before measuring the bleeding time. TXB 2 assay TXB 2 assays were performed using a TXB 2 immunoassay kit obtained from Enzo Lifesciences (UK) and following the manufacturer’s protocols. Briefly, human or mouse PRP was prepared and stimulated with agonists such as CRP-XL in the presence or absence of gap-junction inhibitors (as needed). The samples were centrifuged at 13,000 g for 10 min after aggregation to remove platelets and frozen until required. The levels of TXB 2 in plasma samples were calculated using standard curves. Statistical analysis The data obtained from aggregation, fibrinogen binding, granule secretion and clot retraction assays were analysed using Student’s t -test. Median fluorescence intensity values obtained in fibrinogen binding and granule secretion assays were converted into percentage for comparison of controls with inhibited samples. The tail-bleeding assay data were analysed using the non-parametric Mann–Whitney test using GraphPad Prism (version 5.04) from GraphPad Software Inc. How to cite this article: Vaiyapuri, S. et al . Connexin40 regulates platelet function. Nat. Commun. 4:2564 doi: 10.1038/ncomms3564 (2013).